Visualizing charge separation in bulk heterojunction organic solar cells Solar cells based on conjugated polymer and fullerene blends have been developed as a low-cost alternative to silicon. For efficient solar cells, electron–hole pairs must separate into free mobile charges that can be extracted in high yield. We still lack good understanding of how, why and when carriers separate against the Coulomb attraction. Here we visualize the charge separation process in bulk heterojunction solar cells by directly measuring charge carrier drift in a polymer:fullerene blend with ultrafast time resolution. We show that initially only closely separated (<1 nm) charge pairs are created and they separate by several nanometres during the first several picoseconds. Charge pairs overcome Coulomb attraction and form free carriers on a subnanosecond time scale. Numerical simulations complementing the experimental data show that fast three-dimensional charge diffusion within an energetically disordered medium, increasing the entropy of the system, is sufficient to drive the charge separation process. Plastic solar cells have attracted interest due to their potential to be processed using high-volume low-cost manufacturing techniques resulting in low-cost, low-carbon electricity [1] , [2] . The highest power conversion efficiency reported to date for a single junction polymer based device is 9.2% (ref 3 ). A major improvement in cell efficiency was obtained by the introduction of the bulk heterojunction device (BHJ) structure [4] , [5] consisting of a mesostructured blend film of conjugated polymer and fullerene. Upon light absorption, excitons are produced in the polymer phase and are converted into closely bound electron–hole pairs at the polymer–fullerene interface, sometimes also referred to as charge transfer (CT) states. Here we refer to closely bound charge pairs produced as charge pair states. In an operating solar cell, the bound charge pair states have to dissociate by overcoming the mutual Coulomb attraction between electrons and holes, to form free mobile charges (charge-separated states) that can be extracted as photocurrent. While the dissociation of charge pairs in polymer–fullerene blends has been intensively investigated [6] , [7] , [8] , [9] , [10] , [11] , [12] , [13] , [14] , [15] , [16] , no consensus has yet been reached on how, when and why carriers separate against their mutual Coulomb attraction, to form free independent charges from bound-charge pair states. A point charge description of the electron and hole of the charge pair state appears to result in a high binding energy that would prevent efficient charge separation. Ultrafast initial long-range carrier separation during thermalization of the charge pair states [13] , [16] or delocalization of CT states [9] , [17] , [18] have been proposed to explain the separation mechanism, whereas other researches argue that only the closely separated charge pair states are initially created [19] , [20] , [21] and favourable structural organization is more important than excess energy [13] , [22] , [23] . Recently, ultrafast spectroscopy methods have been employed to follow dynamics of Frenkel-type or CT exciton splitting into charge pairs [7] , [9] , [24] , [25] , [26] . However, these methods are unable to provide information about the electron–hole separation once it exceeds ~1 nm and therefore cannot probe charge carrier escape from the Coulomb field. Direct experimental data on the carrier separation distance during escape from the Coulomb attraction dynamics is required to understand the charge separation process. In this work, we experimentally monitor the carrier separation distance in poly(3-hexylthiophene):phenyl-C61-butyric acid methyl ester (P3HT:PCBM) solar cells with subpicosecond time resolution and visualize how photogenerated bound-charge pairs are separated into free charges, and how subsequently they move in the conjugated polymer:fullerene blend. We use the time-resolved Electric Field-Induced Second Harmonic (EFISH) method [27] , in a pump–probe configuration to probe the electric field dynamics with subpicosecond time resolution. This technique is similar to probing the electric field dynamics by Stark effect [28] , [29] , but the analysis is more straightforward. The dynamics of the electric field allows us to monitor the polarization of molecular charge densities and drift of charge carriers. From the drift dynamics we obtain time-dependent carrier mobility and with the help of the Einstein relation and Monte Carlo (MC) simulations of carrier dynamics, we can resolve the contributions of drift and diffusion to the overall charge separation. This work elucidates charge carrier dynamics on pico-to-nanosecond time scales, filling the knowledge gap left by ultrafast spectroscopic methods that probe excited state dynamics on subpicosecond time scales and electrical methods that probe free carrier motion on nano-to-millisecond time scales. Our measurements allow us to rule out the hypothesis of initial long-range carrier separation. We demonstrate that carrier diffusion alone can account for the separation of the nearest-neighbour interfacial CT state into independent charge carriers. Charge displacement The time dependences of the normalized EFISH signal at various applied voltages are presented in Fig. 1a . The intensity of the EFISH signal measures the reducing electric field inside the blend, as the photogenerated electron and hole charge clouds drift apart, shielding more of the BHJ structure from the applied external field. The field-induced charge pair displacements, that is, sum of drift distances of electrons and holes in opposite directions, extracted directly from the time-dependent EFISH signal at the same applied biases are shown in Fig. 2 (symbols). The charge displacement distances increase on a tens of picosecond time scale. Interestingly, we observe only very small (<1 nm) carrier displacement distances on a subpicosecond time scale. We attribute this modest separation to the field-induced polarization of molecular electron and hole charge densities, similar to exciton polarization observed in neat polymers [27] . It has been established that CT from the polymer to the fullerene acceptor in BHJ blends occurs on a timescale as short as 0.1 ps [9] , [12] . The small charge pair displacement on a subpicosecond time scale shows that the applied electric field has no, or only weak influence on the spatial separation of these nascent bound pair states. This can be understood to be a result of ultrafast formation of nearest-neighbour bound charge pair states with short charge separation distances and varying orientations determined by the varying configurations of the donor:acceptor heterojunctions. This is because even the strongest external electric field in our experiment modulates the Gibbs free energy, driving the formation of nearest-neighbour charge pair states (~0.9 eV; ref. 30 ) by <10%. More widely separated (>5 nm) charge pair states would, on the other hand, be modulated by ~1 eV at strong electric fields and thus be strongly field-dependent, and therefore would be detected in our experiments as large carrier displacements. The absence of a major ultrafast EFISH response therefore leads us to conclude that no long-range charge separation occurs on an ultrafast sub-picosecond timescale. 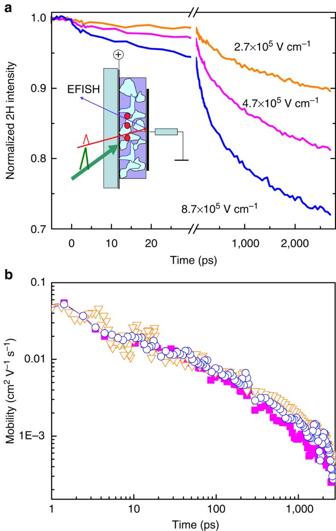Figure 1: Second harmonic kinetics and time-dependent mobility. (a) Experimental kinetics of the second harmonic intensity at different electric field strengths. (b) Time-dependent carrier mobility averaged over electrons and holes determined from experimental data presented in (a). The inset illustrates the measurement scheme. The blend film is situated between ITO and Al electrodes. The electric field was created by the applied external voltage and by different work functions of the electrodes (~0.7 eV). The excitation pulse (green arrow) photogenerates charge carriers, which by drifting partly discharge the capacitor-like sample. The probe pulse, applied after variable delay, is used to monitor the electric field by measuring the second harmonic generation efficiency. Figure 1: Second harmonic kinetics and time-dependent mobility. ( a ) Experimental kinetics of the second harmonic intensity at different electric field strengths. ( b ) Time-dependent carrier mobility averaged over electrons and holes determined from experimental data presented in ( a ). The inset illustrates the measurement scheme. The blend film is situated between ITO and Al electrodes. The electric field was created by the applied external voltage and by different work functions of the electrodes (~0.7 eV). The excitation pulse (green arrow) photogenerates charge carriers, which by drifting partly discharge the capacitor-like sample. The probe pulse, applied after variable delay, is used to monitor the electric field by measuring the second harmonic generation efficiency. 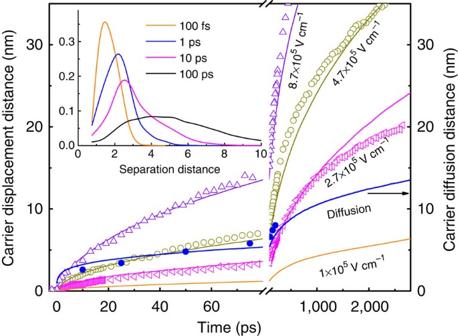Figure 2: Carrier displacement distance. Time-dependent experimental (symbols) and calculated (lines) carrier displacement distance, that is, average charge pair separation distances along the direction of the external electric field of different strength. The electric field is created by the applied external voltage and by different work functions of the electrodes of about 0.7 eV. The solid blue line shows the absolute carrier separation by diffusion at zero electric field obtained from MC simulations, and blue circles show the diffusion distance calculated by the Einstein relation. The inset shows the temporal evolution of the distribution of the absolute carrier separation distances at zero electric field. Full size image Figure 2: Carrier displacement distance. Time-dependent experimental (symbols) and calculated (lines) carrier displacement distance, that is, average charge pair separation distances along the direction of the external electric field of different strength. The electric field is created by the applied external voltage and by different work functions of the electrodes of about 0.7 eV. The solid blue line shows the absolute carrier separation by diffusion at zero electric field obtained from MC simulations, and blue circles show the diffusion distance calculated by the Einstein relation. The inset shows the temporal evolution of the distribution of the absolute carrier separation distances at zero electric field. Full size image Time-dependent mobility Subsequent motion of the charge carriers in the applied electric field may be characterized by a time-dependent effective mobility. We can formally evaluate the instantaneous effective carrier mobility, averaged over electrons and holes, from the experimental kinetics of the carrier displacement distance l(t) at some particular electric field F as . As Fig. 1b shows, the effective mobility decreases gradually on the picosecond-to-nanosecond timescale and is independent of the electric field strength within experimental accuracy. The latter suggests that the charge pair separation is not electric field-dependent in this material system as any field dependence of carrier separation would lead to field dependence of the apparent instantaneous mobility at short times. The initial mobility is at least two orders of magnitude higher than the long-time mobility [31] and is comparable to that obtained in time-resolved terahertz measurements on P3HT:PCBM [32] and other polymer:PCBM blends [33] , [34] . Separation of charges in an electric field has two contributions, field-induced drift (as measured in the present experiments) and diffusion [35] . The diffusion coefficient D is linked to the carrier mobility μ through the Einstein relation (assuming it is valid for organic semiconductors [36] ), where q is the electron charge, k B and T are the Boltzmann coefficient and temperature, respectively. This means that charge carrier drift in any given electric field will be accompanied by a certain amount of diffusion on the same time scale. We use the Einstein relation to calculate the time-dependent diffusion coefficient D(t) from the experimental mobility kinetics presented in Fig. 1 . Next, we use D(t) to obtain a representative distribution of the diffusion distances r as: and hence estimate the average diffusion distance as the peak of this distribution function. This expression accounts for the initial carrier motion in a half space separated by the polymer–PCBM junction and also for an increasing number of available sites as the second power of the separation distance, leading to higher probability for carriers to be separated by larger distances despite the Coulomb attraction opposing separation (see insert in Fig. 2 ). Thus, this entropic factor [37] helps drive the carriers away from their initial positions, while the relaxation of the photogenerated hot carriers to lower energetic levels during diffusion (discussed below) assists this process by making it non-reversible. The inset in Fig. 2 shows the calculated separation distance distributions. The obtained average charge separation distances at different delay times driven by diffusion are presented in Fig. 2 (filled symbols). These results suggest that charges separate rapidly through diffusion: already at 10 ps the peak of the displacement distance distribution is at ~3 nm and a significant fraction of the charges have reached a distance of >5 nm; at 100 ps the majority of the charges have separated to distances exceeding 5 nm by diffusion. We apply a MC model to simulate carrier motion (see Methods ) to examine whether charge carrier diffusion away from the interface in an energetically disordered material is capable of explaining the initial carrier dynamics in the P3HT:PCBM blend. We simulate the experimentally measured carried drift kinetics and obtained diffusion contribution to the total average electron–hole separation distance directly from this numerical experiment. In order to account for the observed time-dependent carrier mobility, the model includes carrier relaxation within a distributed density of states (DOS), as well as motion in a polymer with a networked microscopic structure [38] . The latter feature assumes different carrier hopping rates inside conjugated polymer segments and over barriers between the segments and polymer chains. The Coulomb attraction potential at short distances was approximated as , where is the absolute charge separation distance between electron and hole, ε is the mean permittivity of the material, a is the lattice constant and b is a correction parameter accounting for the smaller charge pair state binding energy (of 0.2 eV (ref. 39 )) than expected from the point charge approximation. We were able to obtain good agreement between experimentally measured and calculated carrier displacement kinetics at different voltages (see Fig. 2 ) with the same set of parameters, changing only the electric field strength. The simulations enable us to determine the diffusion contribution to the charge carrier separation by calculating absolute carrier separation distances at zero applied field. The results in Fig. 2 show that the carrier separation during the initial several picoseconds is dominated by diffusion, which drags charge carriers apart by ~3 nm. The drift starts to contribute more substantially to the carrier separation during the slower ( t >10 ps) phase, but diffusion still strongly dominates at typical electric fields in solar cells (~1 × 10 7 V m −1 ), even on a subnanosecond timescale when the Coulomb electron–hole attraction is effectively overcome (~7–8 nm). The carrier motion slows down rapidly with time as carriers relax into deeper energetic traps within the DOS. Extended polymer segments are also expected to assist the initial charge separation process by allowing carriers to find the fastest transport pathways through the material [33] , [34] . We can now combine the picture of charge diffusion and drift with other features previously suggested to be of importance for facilitating charge separation [9] , [17] . 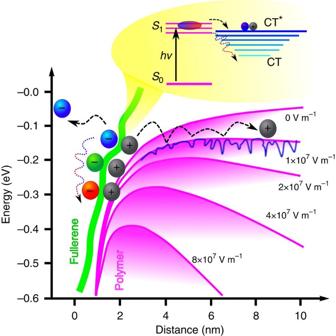Figure 3: Charge carrier separation model. Pink lines show potential surfaces of charge carriers in the vicinity of the counter charge along the applied electric field of different strength, calculated using the point charge approximation. Dashed lines indicate charge motion and the blue line illustrates the potential energy landscape of the disordered polymer. The green line represents the polymer and PCBM interface. Following photoexcitation of the polymer, the manifold of closely bound charge pair states is populated. During the charge separation monitored by the EFISH measurement, the hole on the polymer samples the energy landscape of the polymer and its diffusion coefficient remains high as long as the hole is not trapped in low-energy sites. Successful charge separation occurs when free charges are formed from bound charge pairs by overcoming binding energy through the combined effect of fast diffusion, entropy and relaxation within DOS. Figure 3 illustrates the potential energy surfaces controlling charge separation at various applied voltages, the energetic disorder of the DOS and the polymer potential energy landscape. The progress of the charge separation process within this framework is discussed in some detail in the caption of Fig. 3 . The small polarization of molecular charge densities obtained in the present work is consistent with a small hole delocalization, as suggested in the studies of Bakulin et al . [9] and Deibel et al . [17] This initial displacement is, however, not sufficient to overcome the electrostatic electron–hole interaction; the very fast initial diffusion of unthermalised charges, as revealed by the measured charge displacement here, brings the carriers to a separation distance of ≥5 nm, where the Coulomb interaction is effectively broken, over a time of ~100 ps. This time to convert bound-charge pair states to free mobile charges (charge-separated states) is much shorter than typical geminate charge recombination times (1–100 ns) [12] , explaining the efficient interception of geminate recombination and high yield of separated charges. Figure 3: Charge carrier separation model. Pink lines show potential surfaces of charge carriers in the vicinity of the counter charge along the applied electric field of different strength, calculated using the point charge approximation. Dashed lines indicate charge motion and the blue line illustrates the potential energy landscape of the disordered polymer. The green line represents the polymer and PCBM interface. Following photoexcitation of the polymer, the manifold of closely bound charge pair states is populated. During the charge separation monitored by the EFISH measurement, the hole on the polymer samples the energy landscape of the polymer and its diffusion coefficient remains high as long as the hole is not trapped in low-energy sites. Successful charge separation occurs when free charges are formed from bound charge pairs by overcoming binding energy through the combined effect of fast diffusion, entropy and relaxation within DOS. Full size image In conclusion, by direct observation of the carrier drift dynamics and evaluation of the diffusion rate in a conjugated polymer:fullerene solar cell, we have established that only the nearest-neighbour charge pair states are created at the polymer:PCBM interface on the ultrafast time scale (~100 fs). We visualize how charges separate during the first several picoseconds after photogeneration into still bound pairs with separation distances of several nm, as a result of rapid three-dimensional diffusion. At later times (sub-nanoseconds) they form free mobile charges, mainly as a result of diffusion and to a minor part through drift in the internal electric field in the cell. The experimental results together with simulated carrier dynamics imply that fast carrier motion, for example, along the polymer chain or within ordered polymer stacks, rather than a large initial charge separation distance of charge pairs, is responsible for high dissociation efficiency at typical operating internal electric fields of polymer:fullerene solar cells. Optimization of the material structure directed towards improving the carrier mobility, which governs both the carrier separation and extraction, is one of the important directions to improve the efficiency of polymer:fullerene solar cells. The time-resolved EFISH method has been described in detail elsewhere [27] However, briefly, the applied voltage U appl and difference of work functions of electrodes Δ W , creates an internal electric field in the photovoltaic device, which acts as a parallel plate capacitor, where d is the sample thickness and e is the electron charge. With optical excitation of the device, the pump pulse generates charge carriers; as the charge carriers of different polarities drift apart, they screen the medium from the applied field. We evaluate the electric field strength by using EFISH generation. The EFISH signal is proportional to the square of the internal field [40] . We measure the excitation-induced change of the electric field strength at some particular delay time t by comparing the second harmonic intensity generated in excited, , and not excited, , sample as: . Calculation of l ( t ) Carrier motion leads to a change of the electric field as: , where n is the carrier density, ε and ε 0 are material and vacuum permittivities and is the average carrier displacement distance, that is, the charge separation along the electric field direction induced by the electric field. We determine n from the electrically measured voltage drop over the sample at long times when all created charge carriers are extracted, and it equals to . The time dependence of the average carrier displacement distance is derived as . Devices The active layer in the device was P3HT-blended to 44% by weight with PCBM in chlorobenzene, spun to a thickness of ~115 nm. The hole electrode was ITO with a 45–60-nm layer of PEDOT:PSS spin coated on top, and the electron collecting electrode was aluminium (Al) at a thickness of ~100 nm. The device was made and annealed in a glove box at 140 °C for 30 min and was encapsulated with a glass slide and epoxy. Experimental setup The experimental setup was based on a pump–probe configuration. The laser setup was a 130 fs Ti:sapphire laser operating at 1 kHz. The frequency-doubled (405 nm) pump pulse excites the sample through the glass substrate and ITO electrode. The excitation fluence was 10 12 ph cm −2 pulse −1 , where second-order recombination is insignificant compared with geminate recombination [12] . The probe pulse was obtained using an optical parametric amplifier (TOPAS) tuned to 1,200 nm. The probe beam passes through the adjustable delay line to the sample, where it reflects off the aluminum electrode, and finally is collected by the photomultiplier. The probe beam is P-polarized to have a component of the electric field vector parallel to the applied electric field direction. The second harmonic of the probe pulse generated in the sample is detected by the photomultiplier. A chopper in the pump beam blocks every second pump pulse to measure the second harmonic intensity generated with and without sample excitation, and , respectively. The voltage, creating the electric field in the device, was applied by 10 μs pulses through a 10-kΩ resistance to avoid sample recharging between excitation and probe pulses. The Al electrode was positively biased to avoid charge injection. An oscilloscope was used to measure the photocurrent and to determine the voltage drop at a long delay time, . MC simulation method Charge carrier generation and motion in the P3HT:PCBM blend was modelled by assuming a cubic lattice, with a lattice constant a =1 nm. At short delays, the charge motion is affected by an opposite charge; therefore, the electron and the hole dynamics should be modelled simultaneously. We assume two types of sites representing electron and hole transporting moieties. The lattice is divided into the donor part, where only holes are allowed to reside and the acceptor part for electrons. Simulating the blend structure, the acceptor sites are defined by filling the lattice volume with ellipsoids of identical volumes, but with randomly distributed semi-axes. The ellipsoids are placed at random positions in the lattice. We generate as many ellipsoids as the required proportion between acceptor and donor sites requests. The remaining space in the lattice is filled with donor sites, representing the polymer. The chain length is chosen randomly from the interval [ L −3, L +3], where L is the average chain length set to be 6 nm. A fragment of the final structure can be seen in Fig. 4 . 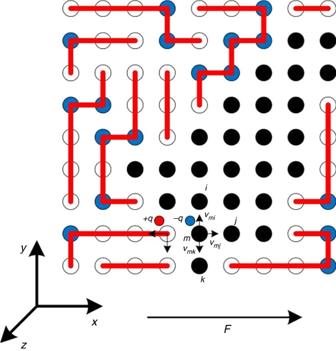Figure 4: Scheme of the model used for the MC calculations. Black dots represent acceptor sites, white dots represent donor sites, blue dots represent folding points of the polymer chains, which are represented by red lines. The external electric fieldFis oriented along thexdirection. Figure 4: Scheme of the model used for the MC calculations. Black dots represent acceptor sites, white dots represent donor sites, blue dots represent folding points of the polymer chains, which are represented by red lines. The external electric field F is oriented along the x direction. Full size image The energy of an electron (hole) in the lattice consists of three parts: (a) internal site self-energy, E r , (b) carrier interaction with electric field, F , and (c) Coulomb interaction with the opposite charge, E C . The electron (hole) energy thus equals to: the site self-energy is distributed according to a modified Gaussian distribution defined as a weighted sum of a normal Gaussian distribution and an exponential distribution extended symmetrically to negative energy values: for electrons and holes, the widths of the distributions are assumed to be different: in the donor part of the lattice (for holes) and in the acceptor part (for electrons). We set the coefficient , implying that the modified Gaussian distribution practically has the shape of an ordinary Gaussian distribution only with the addition of somewhat longer exponential tails. As the initial configuration, the hole and electron are placed on neighbouring sites in the interfacial region of the donor and acceptor domains; only nearest neighbour sites are taken into account for the hopping event. A charge can hop into one of six surrounding sites when it is far from the interface, while hopping possibilities are fewer in the interfacial region. The hopping rates for both electron and hole are calculated using the Miller–Abrahams formula [41] . where γ is a parameter which characterizes the inverse localization length of a charge density, is the distance between the origin site m and the target site n , and and are their energies, respectively. In the acceptor domain is constant, whereas in the donor part we assume for hopping to a target site located in a straight part of the same polymer chaine, for hopping to a target site located on a folding point where orientation of the polymer chain changes, and for hopping to a target site located in a different polymer chain. Carrier motion in a herarchial polymer structure is expresses by difining . The rates are being translated into hopping probabilities according to: where the summation is performed over all calculated rates of both the hole and the electron. These probabilities are used to determine the destination site n for either the hole or the electron, chosen by a linearly distributed random number. The charge configuration is then switched to the one that has been determined and the rates of the next hopping events are recalculated. The time interval between two hops is taken as a random value described by the exponential distribution, characterizing the total hopping rate. In the m -th configuration, the time to reach the m +1-th configuration, , is the random number drawn from: where is the lifetime of the m -th configuration: This determines the time and thus allows to calculate the time-dependent properties. A lattice of 100 × 400 × 400 nm simulates the actual structure of the blend; therefore, no cyclic boundary conditions are introduced. Initially, charges are created at a random location on the interface and due to the external electric field they drift apart in opposite directions. While charges move through the lattice, the distance between them d k ( t ) projected in the direction of the external electric field F is recorded. We assume dielectric permittivities of both materials to be equal to 3. From the fitting procedure the following parameter values were obtained: energy disorder for acceptor and donor materials, 70 and 80 meV respectively, which are close to those determined in the study by Deibel et al . [17] ; hopping rate prefactors in the acceptor, =7.2 × 10 15 s −1 , and in the donor, =3 × 10 16 s −1 , =1 × 10 16 and =3.5 × 10 15 s −1 ; the parameter γ=5 nm −1 . The results were averaged over 5,000 realizations. How to cite this article: Vithanage, D. A. et al . Visualizing charge separation in bulk heterojunction organic solar cells. Nat. Commun. 4:2334 doi: 10.1038/ncomms3334 (2013).